Energy losses of nanomechanical resonators induced by atomic force microscopy-controlled mechanical impedance mismatching Clamping losses are a widely discussed damping mechanism in nanoelectromechanical systems, limiting the performance of these devices. Here we present a method to investigate this dissipation channel. Using an atomic force microscope tip as a local perturbation in the clamping region of a nanoelectromechanical resonator, we increase the energy loss of its flexural modes by at least one order of magnitude. We explain this by a transfer of vibrational energy into the cantilever, which is theoretically described by a reduced mechanical impedance mismatch between the resonator and its environment. A theoretical model for this mismatch, in conjunction with finite element simulations of the evanescent strain field of the mechanical modes in the clamping region, allows us to quantitatively analyse data on position and force dependence of the tip-induced damping. Our experiments yield insights into the damping of nanoelectromechanical systems with the prospect of engineering the energy exchange in resonator networks. For nanoelectromechanical (NEM) resonators [1] , control of vibrational energy exchange between the resonator and its supports is highly desirable: High Q-factor resonators are attained by suppressing this energy transfer [2] , which allows realization of ultrasensitive devices [3] , [4] , [5] , [6] . Conversely, the energy transfer can be engineered to realize integrated resonator devices communicating through phononic waveguides [7] . It is convenient to think of the vibrational modes as localized standing waves caused by the mismatch in mechanical impedance between the support and the suspended region. In this picture, a large impedance mismatch gives rise to a large wave reflection and a correspondingly highly localized vibrational mode with a large Q-factor (limited by internal losses only). To explore the impact of clamping losses [8] on the overall dissipation of a NEM resonator, it may be favourable to modify the mechanical impedance mismatch between resonator and support by a controlled perturbation of the resonator’s acoustic environment. Such a local perturbation can be induced by an atomic force microscope (AFM) tip positioned in the clamping region of the NEM system. AFM based methods have been used with great success to detect the vibrational modes of nanomechanical resonators. In these experiments the investigated mechanical structure is probed by the AFM cantilever, which acts as an active sensing element for the mechanical motion. In such a way, mechanical oscillations have been detected using contact mode AFM [9] , [10] , as well as non-contact techniques [11] , [12] , [13] , [14] . This allowed imaging of the resonator mode shapes and how they are affected by local stress [15] . In addition, a recent study reports the non-linear coupling of two AFM cantilevers of different resonance frequency, enabling the mechanical detection of thermal cantilever motion [16] . In this study, we employ an AFM tip to control the mechanical impedance mismatch between a NEM resonator and its environment. In this complementary approach, inspired by the pioneering work of Topinka et al . [17] , we employ a self-contained NEM system, which is dielectrically driven and detected via an integrated transducer. The AFM is used entirely passively, exerting a controllable perturbation in contact mode. In contrast to the aforementioned schemes, rather than employing the AFM cantilever as a mechanical detector, local perturbation via the AFM tip and the sensitive detection of its impact on the mechanical motion are separated. We use this scheme to obtain insights into the damping of NEM resonators, which to date is not fully understood. The dissipation of the resonator’s flexural modes is found to strongly depend on the position of the tip within the clamping region and follows the evanescent strain field of the mechanical mode in the support. Thus, the presented method of spectroscopy through local mechanical impedance mismatch manipulation yields fundamental insights into the damping of NEM systems. Mechanical impedance mismatch control The NEM system in the focus of this work is a high-Q silicon nitride string resonator, which has been shown to dissipate vibrational energy by energy relaxation into its environment [18] . We show that the local position of the AFM tip on the clamping region of the resonator strongly affects this relaxation pathway. This is reflected in a strong dependence of the resonator damping with the tip position. The observed increase in damping of more than an order of magnitude can be understood by a position-dependent transfer of vibrational energy into the AFM cantilever, which is mediated by minute deformations in its clamping region induced by the resonator’s flexural modes. The amount of transferred energy is independently probed by the decrease in Q-factor of the resonator and controlled by changing the contact position or the force applied to the AFM tip. We find that the effect of the AFM perturbation on the mechanical damping of the resonator is surprisingly large with the tip positioned in the clamping region where the mechanical mode leaks into the support structure. Its impact can suppress a resonance with 35 dB signal to noise ratio below the noise limit. We attribute this observation to the local reduction of the mechanical impedance mismatch between the resonator and its environment. Hence, we are able to study the passage between a highly matched, low-Q system to a highly mismatched, high-Q system on a single resonator, which does not change its internal properties. We theoretically describe this effect with a linear model using Derjaguin–Muller–Toporov theory [19] for the tip–sample interaction as independently suggested by Basarir and Ekinci [16] . We can then quantitatively analyse our data by fitting our model to force-dependent measurements and explain the observed position dependence by comparing our data with finite element simulations of the evanescent strain field of the mechanical modes in the clamping region. While this method does not address all relevant intrinsic sources of damping [20] , [21] , [22] it enables the investigation of the contribution from vibrational modes radiating into the supports [8] , [23] , [24] . AFM and NEM measurement set-up Our experimental set-up ( Fig. 1 ) consists of a high-Q silicon nitride string resonator [25] introduced into an AFM that is operated under vacuum conditions. The resonator ( Fig. 1a ) is dielectrically coupled to two close-lying gold electrodes for both actuation [26] and detection [27] of its dynamics. The fundamental flexural out-of-plane resonance frequency is f 0 ≈6.6 MHz. The room temperature quality factors of the investigated resonators range from Q 0 ≈150,000 to Q 0 ≈250,000, corresponding to damping rates γ 0 =2π f 0 / Q 0 between 277 s −1 and 166 s −1 . 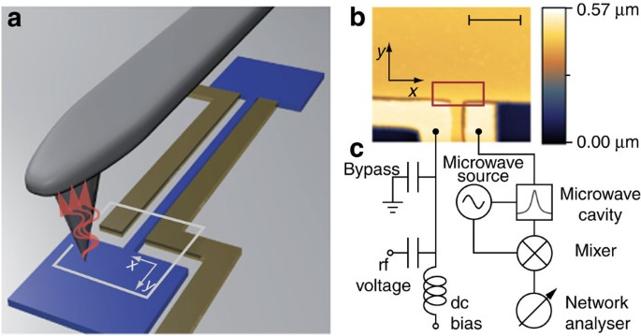Figure 1: Measurement set-up. (a) Illustration of the nanomechanical system with the AFM tip as a controlled local perturbation of the resonator’s acoustic environment. This leads to a flow of energy from the nanomechanical system into the cantilever (grey), as symbolized by the corrugated red arrows. The resonator (blue) is 55 μm long, 250 nm wide and 100 nm thick. It is bordered by two 1 μm wide gold electrodes (yellow) for actuation and detection. The illustration is not to scale to provide better visibility of the individual components. (b) AFM image of a resonator clamp as marked by the light grey frame ina(rotated by 180°). The scale bar corresponds to 2 μm. (c) Electrical set-up. One of the electrodes is connected to a microstrip cavity for detection27, whereas the other electrode is used for the application of an rf voltage and a dc bias for actuation26. The bypass capacitor provides a ground path for the microwave detection35. Figure 1: Measurement set-up. ( a ) Illustration of the nanomechanical system with the AFM tip as a controlled local perturbation of the resonator’s acoustic environment. This leads to a flow of energy from the nanomechanical system into the cantilever (grey), as symbolized by the corrugated red arrows. The resonator (blue) is 55 μm long, 250 nm wide and 100 nm thick. It is bordered by two 1 μm wide gold electrodes (yellow) for actuation and detection. The illustration is not to scale to provide better visibility of the individual components. ( b ) AFM image of a resonator clamp as marked by the light grey frame in a (rotated by 180°). The scale bar corresponds to 2 μm. ( c ) Electrical set-up. One of the electrodes is connected to a microstrip cavity for detection [27] , whereas the other electrode is used for the application of an rf voltage and a dc bias for actuation [26] . The bypass capacitor provides a ground path for the microwave detection [35] . Full size image The AFM is operated in contact mode with constant force. A topographic image of one resonator clamping region is depicted in Fig. 1b . In a typical measurement we use the acquired AFM topography image to define the grid for a point by point measurement in the vicinity of the clamp (red rectangle in Fig. 1b ). The AFM tip is positioned at the first grid point and the driven linear amplitude response of the nanomechanical resonator is measured with a network analyser using the circuitry displayed in Fig. 1c . The topographic information is subsequently read-out and the measurement is repeated on the next grid point. 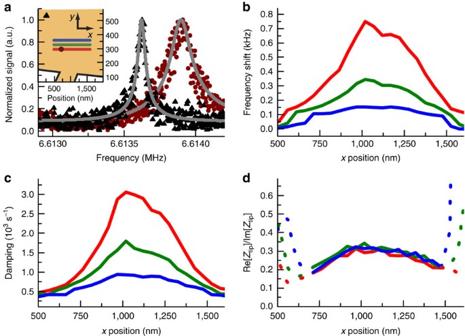Figure 2: Tip-induced frequency shift and damping. (a) Lorentzian amplitude spectra and fits for two spatially well separated tip positions. The inset shows the outlines of the clamping region with the resonator protruding at the bottom (orange,c.f.red rectangle inFig. 1b). The tip positions for the two spectra shown inaare marked with the respective plot marker symbol in the inset. (b) Shift of the resonance frequency with tip position along three lines specified in the inset ofa. The data and the respective tip positions are colour coded. (c) Damping rate versus tip position for the same line cuts. (d) The theoretical model predicts the ratio of real and imaginary parts of the contact impedance to be invariant. This ratio has been computed from the measured frequency shift and damping curves inbandc. As it is only well defined for non-zero frequency shifts and diverges far from the resonator, the dashed sections lie beyond the validity of our model. Tip-induced damping and frequency shift Figure 2 displays the effect of the presence of the AFM tip on the nanomechanical system. The presented data were taken for the fundamental out-of-plane mode of a resonator with an unperturbed resonance frequency f 0 of 6.61 MHz and quality factor Q 0 = f 0 /Δ f 0 of 150,000, where Δ f 0 is the full width at half maximum of the Lorentzian amplitude spectrum, corresponding to a damping rate γ 0 =2πΔ f 0 of 277 s −1 . Normalized amplitude spectra of the resonator for two tip positions in the clamping region, one being close to the resonator (circles) and one farther away (triangles) are depicted in Fig. 2a . The respective tip positions are illustrated in the inset with the respective plot marker symbols. The spectra show a marked shift of the resonance frequency as well as a line broadening. The outline of the clamp also apparent in the inset was extracted from the simultaneously recorded AFM topography data. Note that the convolution of tip shape and sample topography increases the apparent resonator width [28] . For the measurements presented in Fig. 2 , the AFM feedback loop was set to maintain a constant force of 9.2 nN. A Lorentzian fit to each mechanical spectrum yields the respective perturbed resonance frequency f pert and damping rate γ pert =2πΔ f pert for a given tip position. The relative errors for the damping are within the range of a few per cent, whereas the relative errors of the measured frequencies are in the range of parts per million. As these fit errors are small, we plot all data without error bars. Figure 2: Tip-induced frequency shift and damping. ( a ) Lorentzian amplitude spectra and fits for two spatially well separated tip positions. The inset shows the outlines of the clamping region with the resonator protruding at the bottom (orange, c.f. red rectangle in Fig. 1b ). The tip positions for the two spectra shown in a are marked with the respective plot marker symbol in the inset. ( b ) Shift of the resonance frequency with tip position along three lines specified in the inset of a . The data and the respective tip positions are colour coded. ( c ) Damping rate versus tip position for the same line cuts. ( d ) The theoretical model predicts the ratio of real and imaginary parts of the contact impedance to be invariant. This ratio has been computed from the measured frequency shift and damping curves in b and c . As it is only well defined for non-zero frequency shifts and diverges far from the resonator, the dashed sections lie beyond the validity of our model. Full size image Both the frequency shift δf = f pert − f 0 and the damping γ pert for tip positions following the three traces depicted in the inset of Fig. 2a are displayed in Fig. 2b,c , respectively. The separation between the traces of 40 nm largely exceeds the estimated diameter of the contact area, which is of the order of about 5 nm for a typical tip. The measurements clearly show a position-dependent shift of the resonance frequency to higher frequencies as well as an increase in damping rate as the tip is brought into the vicinity of the clamping region. Remarkably, even for the tip at a distance of 150 nm from the freely suspended part of the resonator ( c.f. centre of the red trace in Fig. 2c ) the tip-induced energy extraction already increases the damping rate by more than an order of magnitude from the unperturbed value. This reduces the quality factor of the resonance from 150,000 to a value below 2,000 before it vanishes in the noise floor. Modelling the mechanical impedance We theoretically describe this effect in a lumped element model, in which the effect of the AFM tip pressing down at a location x 0 in the clamping region is modelled as an additional mechanical impedance (hereafter referred to as contact impedance) For the n -th ( n =0, 1, 2, …) eigenmode of the resonator, the frequency-dependent linear amplitude response to an external driving force can then be written as with being the effective resonator mode mass given by integrating over the square of the normalized resonator amplitude ( x ), that is, the amplitude of the local surface deformation divided by its maximum value at an antinode of the string. Here ω n =2π f n and γ n are the free resonance frequency and damping rate of the n -th mode ( n =0, 1, 2, …). Derivations of equations (1) and (2) can be found in the Supplementary Methods . The contact impedance Z tip for the n -th mode depends on position through ( x 0 ). Its frequency dependence is contained in the function describing the motion of the cantilever tip in response to force exerted on it by the vibrating surface. We describe the force-dependent coupling constant g within the Derjaguin–Muller–Toporov theory [19] (see Supplementary Methods for details). The real and imaginary parts of Z tip relate to the additional damping and the frequency shift via Re[ Z tip ]= m n δγ = m n ( γ pert − γ n ) and Im[ Z tip ]=2 m n δω =2 m n ( ω pert − ω n ), respectively. The former arises from vibrational energy that is transmitted into the AFM cantilever and dissipated there while the latter is a result of modified wave reflection. Equation (1) is derived assuming a linear relation between the force on the cantilever tip and its motion. It is apparent from equation (1) that the ratio of real and imaginary parts should be independent of tip position x 0 . The corresponding data for the fundamental out-of-plane mode ( n =0), which are displayed in Fig. 2d , confirm this expectation, even though a slight curvature visible in the data cannot be accounted for using a linear model. We additionally conducted a measurement for the third harmonic of the out-of-plane mode ( n =2) and found the same behaviour with similar numerical values (see Supplementary Methods ). Force-dependent measurements The force dependence of Z tip , contained in the coupling g in equation (1) was studied by recording force–distance curves at different tip positions. As the local normalized resonator amplitude ( x 0 ) varies for these positions, so do the frequency shift and the induced damping for a given force. In the linear theory, however, all curves can be scaled to coincide. Thus, an entire data set for frequency shift and damping at multiple positions can be fitted with a single set of parameters. 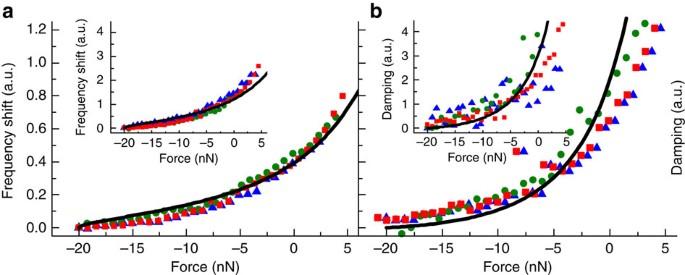Figure 3: Force dependence of frequency shift and damping. Force–distance curves are measured at three points in the clamping region (red squares, green dots, blue triangles) with increasing distance to the resonator. Since a linear response theory is valid, all curves can be scaled to coincide with each other. Thus, our model can be fitted to the whole data set, that is, all frequency shift and damping curves, with one single set of parameters. For clarity, we only show the retraction curves. In all panels red squares represent the data for the point of highest interaction (closest to the clamp), green dots for an intermediate and blue triangles for the point of lowest interaction. (a) Force dependence of the frequency shift of the fundamental out-of-plane mode with a free resonance frequency of 6.65 MHz. The solid black line is a fit of the model. The inset shows the data and fitted model of the third harmonic mode with a free resonance frequency of 20.0 MHz, which was measured simultaneously. (b) Force dependence of the tip-induced damping for the same modes. Figure 3 shows the fit of our model to the experimental data for a resonator with an unperturbed resonance frequency of f 0 =6.65 MHz and damping rate of γ 0 =173 s −1 . Here the force–distance curves were measured for three different tip positions in the clamping region, indicated by colour (not related to the colour coding of Fig. 2 ). The rescaled data show very good quantitative agreement with the model, confirming the validity of the linear approach (see Supplementary Methods for details on the fitting procedure and the resulting fitting parameters). Figure 3: Force dependence of frequency shift and damping. Force–distance curves are measured at three points in the clamping region (red squares, green dots, blue triangles) with increasing distance to the resonator. Since a linear response theory is valid, all curves can be scaled to coincide with each other. Thus, our model can be fitted to the whole data set, that is, all frequency shift and damping curves, with one single set of parameters. For clarity, we only show the retraction curves. In all panels red squares represent the data for the point of highest interaction (closest to the clamp), green dots for an intermediate and blue triangles for the point of lowest interaction. ( a ) Force dependence of the frequency shift of the fundamental out-of-plane mode with a free resonance frequency of 6.65 MHz. The solid black line is a fit of the model. The inset shows the data and fitted model of the third harmonic mode with a free resonance frequency of 20.0 MHz, which was measured simultaneously. ( b ) Force dependence of the tip-induced damping for the same modes. Full size image Impedance maps To further investigate the dependence of the contact impedance Z tip on the local normalized resonator amplitude ( x 0 ) we recorded impedance maps for the fundamental ( n =0) out-of-plane and in-plane mode of the resonator and compared the data with COMSOL finite element simulations of (out-of-plane) and (in-plane) ( Fig. 4 ). Again, the measurements were conducted on a grid of tip positions in the vicinity of the resonator clamping region with the AFM tip exerting a constant force. The contact impedances were then calculated from the induced damping Re[ Z tip ]= m n δγ and the frequency shift Im[ Z tip ]=2 m n δω . The data for the out-of-plane mode ( Fig. 4a,b ) stem from the same measurement as the frequency shift and damping presented in Fig. 2 . The real part of the contact impedance for the in-plane mode presented in Fig. 4c was measured on a different resonator with an unperturbed resonance frequency of 6.82 MHz, a damping rate of 357 s −1 and zero cantilever deflection. 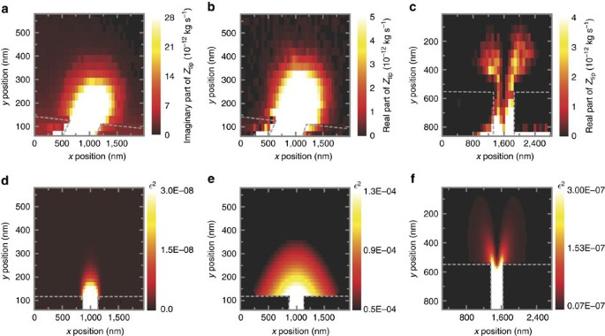Figure 4: Impedance maps. Experimentally determined contact impedance maps (a–c) and simulated local amplitudes of the clamping region (d–f) for the fundamental out-of-plane and in-plane mode. (a) Imaginary part of the contact impedanceZtipfor the out-of-plane mode. (b) Real part of the contact impedance for the out-of-plane mode. (c) Real part of the contact impedance for the in-plane mode. (d) Simulated normalized squared amplitudefor the out-of-plane mode for a clamp with no undercut. (e) The same with a realistic undercut of the silicon nitride pedestal of 500 nm. (f) Simulatedfor the fundamental in-plane mode with 500 nm undercut. Figure 4: Impedance maps. Experimentally determined contact impedance maps ( a – c ) and simulated local amplitudes of the clamping region ( d – f ) for the fundamental out-of-plane and in-plane mode. ( a ) Imaginary part of the contact impedance Z tip for the out-of-plane mode. ( b ) Real part of the contact impedance for the out-of-plane mode. ( c ) Real part of the contact impedance for the in-plane mode. ( d ) Simulated normalized squared amplitude for the out-of-plane mode for a clamp with no undercut. ( e ) The same with a realistic undercut of the silicon nitride pedestal of 500 nm. ( f ) Simulated for the fundamental in-plane mode with 500 nm undercut. Full size image Comparing the spatial contact impedance profiles ( Fig. 4a–c ) with the simulated local resonator amplitudes displayed in Fig. 4d–f convincingly shows that the experimental data can be accurately reproduced by the simulations. It is thus possible to image the evanescent decay of the local strain field of the respective mechanical mode as it leaks into the clamping region. This also explains the strong spatial dependence of the additional damping away from the contact (y-direction in Fig. 4 ) as such a decay generally depends exponentially on position. In that sense, the energy transfer into the AFM cantilever can also be interpreted as a frustrated internal reflection of the mechanical wave incident at the clamping point. However, the exact shape of the decaying amplitude profile strongly depends on the microscopic clamping region geometry. Since the last step of the fabrication process is an isotropic hydrofluoric wet etch of the fused silica substrate to obtain freely suspended strings [27] , a small part of the clamp becomes underetched as well. This in turn has a large effect on the local amplitude, which is demonstrated for the out-of-plane mode in Fig. 4d,e . Figure 4d shows the simulated for a clamp with no undercut, giving rise to a quickly decaying strain field. Figure 4e in turn was simulated with a realistic, 500 nm deep undercut, yielding excellent qualitative agreement with Fig. 4b . Since the in-plane mode oscillates within the substrate plane, the resulting amplitude profile drastically differs from the out-of-plane mode. For reasons of symmetry, the in-plane profile exhibits a node with zero displacement along the symmetry axis—analogous to the neutral surface in a bent beam ( Fig. 4c ). Figure 4f displays the simulated local amplitude of the in-plane mode, again excellently corresponding with the measured data. Lastly, to indicate the displacement of the surface at the position of the AFM tip, we make the following estimation: From a calibration via the resonator’s brownian motion [27] we find that typical maximum amplitude values in our measurements are of the order of 6 nm. From the force-dependent measurements we can calculate the surface displacement at the tip position using the obtained ( x ). The smallest ε value is =2.1 × 10 −4 , so that the estimated maximum surface displacement d max at this point is d max =6 nm × 2.1 × 10 −4 =1.26 pm. For the in-plane mode, the resonator amplitudes are of the same order. The simulations yield ε values as small as =1 × 10 −4 (compare Fig. 4d ), so that here the surface amplitudes can be estimated to be as small as ≈0.6 pm. In summary, we present a method of locally controlling the mechanical impedance mismatch of a NEM resonator and its environment, which offers valuable insight into the damping behaviour of resonant elements. Altering the contact impedance mismatch by means of an AFM tip interacting with the mechanical strain profile extending into the resonator clamping region changes the amount of energy that is radiated into the resonator’s environment [24] and results in a striking change in Q-factor. As the intrinsic damping of the resonator remains unchanged in the experiment, the tip-position-dependent induced damping is a direct measure of the mechanical damping resulting from radiation losses. Such radiation losses, commonly referred to as phonon tunnelling [8] , are a much discussed damping mechanism in the field of nanomechanics [2] , [23] , [24] , [29] , [30] , [31] , [32] , [33] . In our experiments we thus show how radiation of vibrational energy into the environment can become the dominant damping mechanism for a NEM resonator. Imaging of the contact impedance in the clamping region then enables mapping of the surface profile of the mechanical mode leaking into the support structure with nanometre lateral resolution. Comparing the experimental data with finite element simulations and studying simulations of structures without undercut shows how the microscopic geometry of the clamping region has a considerable influence on the evanescent decay of the mode and hence on the impedance mismatch of the mechanical device. Even though the Q-factors of our resonators are not yet limited by clamping losses [21] , a further improvement of high Q-factor structures will require careful engineering of the mechanical impedance mismatch. The presented scheme could prove to be a valuable tool for this endeavour. Moreover, the force dependence of the contact impedance is very interesting for investigations of tip–sample interactions, as substantial surface forces are exerted while maintaining a linear interaction regime. Finally, an exciting application for this new method of mechanical impedance spectroscopy lies in the development of integrated nanomechanical networks, since control over the mechanical impedance matching is vital [2] , [7] , [34] for the energy confinement and exchange between resonant structures and thus for future applications of NEM. Atomic force microscope The employed AFM is an attoAFM I , manufactured by attocube systems. It uses a fibre interferometric read-out of the cantilever deflection and is suited for vacuum operation. All measurements are carried out inside the vacuum chamber of this device at pressures of <10 −4 mbar and room temperature. To allow the utilization of the microwave detection scheme [27] , the AFM was additionally equipped with microwave cabling. A hand-formable cable (Micro-Coax UT-85C-FORM) is used to connect an SMA vacuum feedthrough to a semi rigid cable (Micro-Coax UT-85B-SS). The semi rigid cable leads to ~15 cm above the sample holder. From here a flexible cable (RG-178/U) is used to transfer the microwave signal to the sample holder. This allows to transfer the microwave signal to the sample holder with relatively small damping (≈5 dB along the set of cables) while maintaining AFM operability by not exerting too large a load on the AFM piezo scanning stage. We employed contact mode silicon cantilevers (BudgetSensors ContAl , 450 μm long, 50 μm wide and 2 μm thick) with force constants around 0.2 N m −1 for all measurements. The only exception is the measurement of the in-plane mode in Fig. 4c , which was conducted with a triangular silicon nitride cantilever manufactured by Veeco (DNP-S10). Sample fabrication All our resonators are fabricated on 500 μm thick fused silica wafers, which are coated with a 100 nm thick commercial LPCVD layer of strongly pre-stressed silicon nitride. To enable electron-beam lithography on the insulating substrate, 3 nm of chromium is evaporated onto the PMMA resist before exposure and removed before developing. Both the gold electrodes and a thin cobalt etch mask protecting the strings are defined in two subsequent electron-beam lithography steps followed by metal evaporation and lift-off. As a next step, an inductively coupled plasma reactive ion etch using SF 6 and Ar removes the silicon nitride which is not protected by a gold or cobalt cover. Finally, a hydrofluoric acid wet etch removes the cobalt etch mask and simultaneously releases the beams. The gold electrodes are processed with a chromium adhesion layer, which is not attacked by the acid. As a last step, the chips are wire bonded to the read-out microwave cavity. How to cite this article: Rieger, J. et al . Energy losses of nanomechanical resonators induced by atomic force microscopy-controlled mechanical impedance mismatching. Nat. Commun. 5:3345 doi: 10.1038/ncomms4345 (2014).